Vanadium dioxide nanowire-based microthermometer for quantitative evaluation of electron beam heating Temperature measurement is critical for many technological applications and scientific experiments, and different types of thermometers have been developed to detect temperature at macroscopic length scales. However, quantitative measurement of the temperature of nanostructures remains a challenge. Here, we show a new type of microthermometer based on a vanadium dioxide nanowire. Its mechanism is derived from the metal–insulator transition of vanadium dioxide at 68 °C. As our results demonstrate, this microthermometer can serve as a thermal flow meter to investigate sample heating from the incident electron beam using a transmission electron microscope. Owing to its small size the vanadium dioxide nanowire-based microthermometer has a large measurement range and high sensitivity, making it a good candidate to explore the temperature environment of small spaces or to monitor the temperature of tiny, nanoscale objects. The rapid development of nanotechnology increases the urgency for developing more accurate and precise quantitative measurement capabilities of small-scale interactions. To date, robust solutions for quantitative measurement of local temperature and heat flow at nanoscale dimensions are very limited [1] , [2] , [3] , [4] , [5] , [6] , [7] , [8] . In particular, inhomogeneous temperature distributions at these size scales are not easily probed with typical small-scale thermal measurements such as infrared thermometers or scanning thermal microscopy [2] , [8] . A primary example of this type of inhomogeneous temperature distribution is the temperature rise in a specimen due to the incident electron beam in a transmission electron microscope (TEM) [9] . In addition to damage mechanisms from high-energy electrons such as knock-on damage, ionization and radiolysis, heating from the electron beam can be particularly important in materials with low thermal conductivity or sample geometries, such as nanoparticles with inadequate thermal contact to the substrate [9] , [10] . Typically, a theoretical estimation can be made for the energy loss of the incident electron beam [10] , but experimentally this interaction is seldom measured. Experimentally, scanning thermal microscopy [2] requires a complicated setup, which is difficult to combine with TEM. The melting point of a material can be used to quantify temperature, but this is typically only a single-point or single-temperature detection [4] , [5] , [6] , [7] , especially when trying to measure the temperature of individual small particles. As environmental interactions become more accessible through modern in situ TEM instrumentation, it is essential to distinguish temperature effects from other electron beam effects [11] , [12] . Here, we demonstrate a new type of microthermometer based on a VO 2 nanowire (NW), which derives its fundamental sensing mechanism from the well-known metal–insulator transition in VO 2 at 68 °C (refs 13 , 14 , 15 ). Using this new type of microthermometer, we can not only measure the temperature of small structures but also the heat flow rate generated by a local interaction with the NW, such as the bombardment of high-energy particles. Temperature measurement with VO 2 NW As shown in Fig. 1a , a 59.8-μm-long VO 2 NW with a cross-sectional area of 0.20 μm 2 was transferred onto a Cu TEM grid using a micromanipulator (Omniprobe) in a focused ion beam (FIB). Following this, a 34.5-μm-long Si NW with a cross-sectional area of 0.31 μm 2 was mounted on top of the VO 2 NW. At the joints of both the TEM grid and VO 2 NW and the Si NW and VO 2 NW, electron beam-induced Pt was deposited to join them together, as shown in Fig. 1b schematically. All of the thermal measurements were carried out in a JEOL 3010 TEM, where the electron beam acted as the local heat source. Owing to the vacuum of the TEM column, heat convection can be ignored [16] and radiation contributions are also safely negligible, as calculated in the Supplementary Note I . 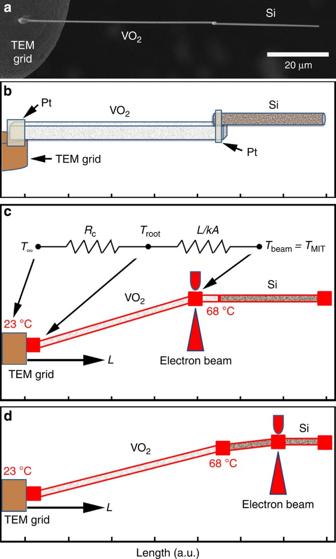Figure 1: Temperature measurement using a VO2and Si nanowire in a TEM. (a) Scanning electron microscope picture of the VO2NW cantilever, extending from the TEM grid, on top of which a Si NW was mounted. (b) Schematic of the setup ina, showing the location of the electron beam-deposited Pt joints. (c) Diagram of the thermal resistance from the TEM grid to the region under the electron beam and schematic of the temperature distribution within the NWs, when the electron beam was located on VO2NW. (d) Schematic of the temperature distribution within the NWs when the electron beam was located on Si NW. Therefore, our analysis can be limited to one-dimensional thermal conduction so that the heat flow rate through the NWs follows the Fourier law, Figure 1: Temperature measurement using a VO 2 and Si nanowire in a TEM. ( a ) Scanning electron microscope picture of the VO 2 NW cantilever, extending from the TEM grid, on top of which a Si NW was mounted. ( b ) Schematic of the setup in a , showing the location of the electron beam-deposited Pt joints. ( c ) Diagram of the thermal resistance from the TEM grid to the region under the electron beam and schematic of the temperature distribution within the NWs, when the electron beam was located on VO 2 NW. ( d ) Schematic of the temperature distribution within the NWs when the electron beam was located on Si NW. Full size image where the thermal conductivity of VO 2 is k VO 2 ≈4.1±0.9 Wm −1 K −1 (see Supplementary Note II ), A is the cross-sectional area, T beam is the temperature of the NW under the electron beam, T root is the temperature of the NW root where it meets the TEM grid and L is the NW length between the root and region under the electron beam. It should be noted that the cross-sectional area is measured using the scanning electron microscope during sample preparation. It is important to emphasize that, since the NW was very small compared with millimetre-sized TEM grid that the heat flow from the NW was too insignificant to change the grid temperature. Furthermore, as the joint thermal resistance was small enough to be neglected (as discussed in detail later), the NW root can be considered to have the same temperature as the TEM grid, which we take as the room temperature of T ∞ =23 °C. The temperature measurement concept is then based on the fact that as more and more electrons are focused on the extended part of the VO 2 NW, the temperature of the local region becomes higher and higher, until the metal–insulator transition (MIT) occurs at 68 °C. The phase transition can be clearly observed in diffraction patterns of the pristine monoclinic I phase (M1) VO 2 and the phase-transformed rutile phase (R) VO 2 at high temperature in Fig. 2a,b . At steady state, the heat flows from the higher-temperature part of the NW (under the electron beam) to the lower-temperature part (attached to the TEM grid), resulting in a temperature distribution shown schematically in Fig. 1c . The electron beam location can be varied along the length of the NW, with the temperature fixed at the region under the beam and the NW root, T beam =68 °C and T root ≈ T ∞ =23 °C, respectively. The heat flow rate generated by the electron beam irradiation is dependent on the location of the electron beam through L as described by the equation (1). 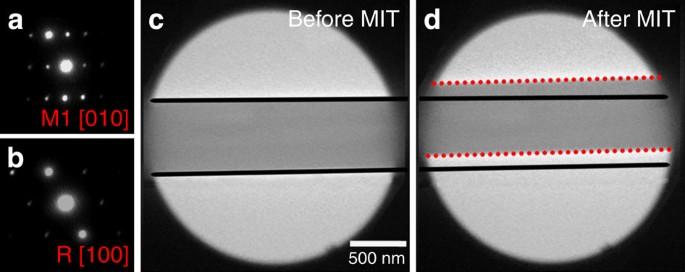Figure 2: Phase transition of VO2nanowire in the TEM. (a) Electron diffraction pattern of the M1 phase of the VO2NW before the phase transition, zone axis [010]. (b) Electron diffraction pattern of the VO2NW in the R phase after the phase transition, zone axis of [010]. From the diffraction patterns the phase transition in VO2could be observed directly. (c) TEM bright field image of the Si NW before the VO2phase transition. (d) TEM bright field image of the Si NW after VO2phase transition. As indicated by the red dashed line, the Si NW moved suddenly from the previous position indicated by the black line, due to the MIT-induced mechanical motion. Therefore, the VO2phase transition could be detected even when electron beam was on Si NW, but not on VO2NW. Figure 2: Phase transition of VO 2 nanowire in the TEM. ( a ) Electron diffraction pattern of the M1 phase of the VO 2 NW before the phase transition, zone axis [010]. ( b ) Electron diffraction pattern of the VO 2 NW in the R phase after the phase transition, zone axis of [010]. From the diffraction patterns the phase transition in VO 2 could be observed directly. ( c ) TEM bright field image of the Si NW before the VO 2 phase transition. ( d ) TEM bright field image of the Si NW after VO 2 phase transition. As indicated by the red dashed line, the Si NW moved suddenly from the previous position indicated by the black line, due to the MIT-induced mechanical motion. Therefore, the VO 2 phase transition could be detected even when electron beam was on Si NW, but not on VO 2 NW. Full size image To quantify the heat flow, we apply steady-state energy conservation to a control volume surrounding the region where the electron beam hits the NW. For beam current I and accelerating voltage V , the maximum heating power that could be deposited if the beam were fully thermalized is P = IV . Note that here and throughout this analysis, I represents only the current incident on the sample, and has been scaled from the total beam current of the TEM spot size using the sample area fraction in each image. On average, however, each incident electron only loses a small fraction of its kinetic energy, with typical inelastic energy losses of order ~100 eV (ref. 10 ). To quantify this effect, we introduce a dimensionless energy absorption coefficient, α , defined as the ratio of the absorbed heating power to the power of the incident beam (0≤ α ≤1). This definition is consistent with the concept of an absorption coefficient as used in radiation heat transfer. Thus the heat conducted away from the beam focal spot is Therefore, by combining equations (1) and (2), we find We apply this result to the experiment on the VO 2 NW shown schematically in Fig. 1c , when the temperature under the electron beam just reaches the phase transition temperature of 68 °C. The results of the beam current needed to achieve the MIT phase transformation as a function of beam position are shown in Fig. 3a . The result is α VO 2 =6.8 × 10 −4 , corresponding to an average energy loss of around 200 eV per electron. Thus, ~1 to ~3 μW of heat is deposited by the incident electron beam into the VO 2 NW, as shown in Fig. 3b . Note that this value of 200 eV describes the overall net energy transfer from the primary electron beam to the sample, and cannot distinguish the individual effects of transmission, secondary electron emission, X-ray emission and so on [10] ; but these effects also do not separately impact the local temperature rise of the solid material, as it is only the total net energy deposition that matters. 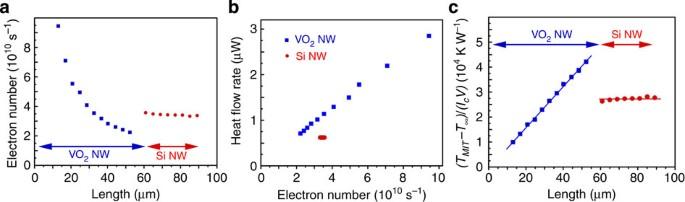Figure 3: Experimental measurement of heat flow through Si and VO2nanowires. (a) Plot of the number of electrons illuminating the NW that are required to trigger the phase transition in VO2NW as a function of electron beam positionL. (b) Heat flow rate generated from the electron beam irradiation on the VO2NW and Si NW. (c) Plot of the combined thermal model of equations (4) and (5) (lines), showing very good agreement with the experimental data (points), and verifying the energy absorption coefficients are essentially constant within the VO2(αVO2≈6.8 × 10−4) and Si (αSi≈3.8 × 10−4), respectively. The intercept atL=0 is essentially zero, confirming that the contact resistance between the TEM grid and VO2NW is indeed negligible. Figure 3: Experimental measurement of heat flow through Si and VO 2 nanowires. ( a ) Plot of the number of electrons illuminating the NW that are required to trigger the phase transition in VO 2 NW as a function of electron beam position L . ( b ) Heat flow rate generated from the electron beam irradiation on the VO 2 NW and Si NW. ( c ) Plot of the combined thermal model of equations (4) and (5) (lines), showing very good agreement with the experimental data (points), and verifying the energy absorption coefficients are essentially constant within the VO 2 ( α VO 2 ≈6.8 × 10 −4 ) and Si ( α Si ≈3.8 × 10 −4 ), respectively. The intercept at L =0 is essentially zero, confirming that the contact resistance between the TEM grid and VO 2 NW is indeed negligible. Full size image Temperature measurement with Si NW When the electron beam is moved onto the Si NW as shown schematically in Fig. 1d , a phase transition in VO 2 was still expected at large beam currents. In this case, since electron beam was on the Si NW, the MIT in VO 2 NW could not be observed directly. On the basis of the previous research [17] , it is known that the MIT induces a change in shape corresponding to a shrinking of the NW by 1% during MIT. Here, this shape change could be seen as an abrupt lateral jump of the Si and was used as an indication of the MIT (as shown in the Fig. 2c,d and Supplementary Movie 1 ). For undoped and strain-free VO 2 NW, the MIT must start at the region of highest temperature, which in this case would be right at the Si NW–VO 2 NW joint. Figure 1d shows the schematic temperature distribution when a high-enough electron beam current was focused onto the Si NW to heat the Si NW–VO 2 NW joint to 68 °C. When the electron beam hit on different regions of Si NW triggering the phase transition in VO 2 , the heat flow rate was constant due to the fixed temperature at both ends of the whole VO 2 NW, as described by the equation (1). Thus the heat flow rate, 0.62 μW, is independent of the electron beam position on the Si NW. The principal feature of this model is now the L independence of I for L >60 μm, which is verified in Fig. 3c to very good agreement. Thus the conversion efficiency α Si is 3.8 × 10 −4 (corresponding to 110 eV per electron). The fact that α Si < α VO 2 indicates that the electron beam has stronger inelastic interactions with VO 2 than Si in our experiments. This is consistent with the fact that in principle, the average scattering section in VO 2 is larger than in Si (ref. 9 ). However, it is important to recognize that α also depends on the material, sample geometry (especially thickness and orientation) and beam voltage, which were not investigated systematically here. It is important to consider the effect of the thermal contact resistance at the joint between the VO 2 NW and the Cu TEM grid and also the joint between the VO 2 NW and Si NW. To do so, we allow for a contact resistance R c between the base of the VO 2 NW at T root and the heat sink T ∞ (shown schematically in Fig. 1c ). This R c accounts for any temperature drop through the Pt bonding as well as heat spreading resistance within the supporting TEM grid. In series with R c is the conduction resistance of the VO 2 NW itself, L / kA . Any offset errors in defining L will be taken into account by R c . For various values of L we consider the critical beam current I c required to just reach the phase transition temperature at the beam spot. From the thermal resistance network we have . Substituting from equation (2) Thus, a plot of versus L (for the I c where T beam = T MIT ) has a slope that reveals α VO 2 and an intercept related to R c . As shown in Fig. 3c , the linear fit of this plot is excellent, with a slope of 823 KW −1 μm −1 . The intercept is essentially zero, confirming that the contact resistance R c is indeed negligible (due to experimental uncertainties, the fit intercept actually takes a slightly negative value of ≈0.065 × 10 4 KW −1 ). Finally we consider the heat flow when the electron beam is incident on the Si NW. In this case, the sample jump occurs when the hottest portion of the VO 2 NW just reaches MIT, regardless of any additional temperature rise in Si. Again neglecting radiation losses, this means that I c is independent of the location of the electron beam within the Si NW. We now find where we have also used the fact that the R C between the VO 2 and the base can be neglected. The principal feature of this model is now the L independence of I c for L >60 μm, which is verified in Fig. 3c to very good agreement (r.m.s. residual error <2%). The average value of is 2.73 × 10 4 KW −1 , used with equation (5) to calculate the value of α Si given above. Having demonstrated this microthermometer’s unique ability to measure electron absorbtion coefficients α , we now consider further broadening its range of use. Since the threshold temperature of the MIT was found previously [18] , [19] to be tunable by doping of the VO 2 NW with W, this general microthermometer measurement method is not limited to only temperatures above 68 °C. As such, the setup could be modified to detect temperatures lower than the MIT temperature. In this regard, the measurement range is in theory variable and spans a wide temperature range since it is possible to measure a temperature distribution. In addition, the size of the microthermometer could be made to be thinner than 100 nm, which would increase its sensitivity to better than 1 °C. Further, it is possible to see the phase transformation using optical microscopy and thus this type of microthermometer is not limited to electron microscopes for sensing. In summary, we reported a new type of microthermometer based on a VO 2 NW that can quantitatively investigate the electron beam heating effect on Si and VO 2 NWs using a transmission electron microscope. We demonstrated that the thermal contact resistance is negligible and using a simple conduction heat transfer model could determine the heat flow rate and energy absorption coefficient of electron irradiation on the Si and VO 2 NWs. Using the mechanical response and visualization of a well-known solid–solid phase transformation, this type of microthermometer should be adaptable for use over a wide temperature range and not limited to only be used in electron microscopes. NW preparation and thermometer assembly The VO 2 NWs were synthesized using the vapour transport method. Si NWs were fabricated on a Si wafer with gold nanoparticles as the catalysts. A free-standing VO 2 NW was transferred onto a Cu TEM substrate, and the Si NW was attached on the top of the VO 2 NW using an Omniprobe manipulator in FEI Dual Beam FIB. Electron beam-induced Pt deposition was used to bond the Si and VO 2 NWs, as well as the VO 2 NW and substrate together. Following this sample preparation, the temperature measurement experiments were conducted in a JEOL 3010 TEM. How to cite this article: Guo, H. et al. Vanadium dioxide nanowire-based microthermometer for quantitative evaluation of electron beam heating. Nat. Commun. 5:4986 doi: 10.1038/ncomms5986 (2014).